Millisecond charge-parity fluctuations and induced decoherence in a superconducting transmon qubit The tunnelling of quasiparticles across Josephson junctions in superconducting quantum circuits is an intrinsic decoherence mechanism for qubit degrees of freedom. Understanding the limits imposed by quasiparticle tunnelling on qubit relaxation and dephasing is of theoretical and experimental interest, particularly as improved understanding of extrinsic mechanisms has allowed crossing the 100 microsecond mark in transmon-type charge qubits. Here, by integrating recent developments in high-fidelity qubit readout and feedback control in circuit quantum electrodynamics, we transform a state-of-the-art transmon into its own real-time charge-parity detector. We directly measure the tunnelling of quasiparticles across the single junction and isolate the contribution of this tunnelling to qubit relaxation and dephasing, without reliance on theory. The millisecond timescales measured demonstrate that quasiparticle tunnelling does not presently bottleneck transmon qubit coherence, leaving room for yet another order of magnitude increase. Quasiparticle (QP) excitations adversely affect the performance of superconducting devices in a wide range of applications. They limit the sensitivity of photon detectors in astronomy [1] , [2] , the accuracy of current sources in metrology [3] , the cooling power of micro-refrigerators [4] and could break the topological protection of Majorana qubits [5] . In superconducting quantum information processing (QIP), the preservation of charge parity (even or odd number of electrons) has historically been a primary concern. In the first superconducting qubit, termed the Cooper-pair box (CPB) [6] , maintaining the parity in a small island connected to a reservoir via Josephson junctions is essential to qubit operation. The qubit states |0〉 and |1〉 consist of symmetric superpositions of charge states of equal parity, brought into resonance by a controlled charge bias n g and split by the Josephson tunnelling energy E J ( ≲ E C , the island Cooper-pair charging energy). QP tunnelling across the junction changes the island parity, ‘poisoning’ the box until parity switches back or n g is offset by ± e (ref. 7 ). QP poisoning has been extensively studied in CPBs and similar devices, such as single-Cooper-pair transistors and charge pumps, with most experiments [8] , [9] , [10] , [11] , [12] , [13] finding parity switching times of 10 μs–1 ms, and some >1 s (refs 14 , 15 , 16 ). While these times are long compared with qubit gate operations ( ∼ 10 ns), the sensitivity of the CPB qubit transition frequency ω 01 to background charge fluctuations limits the dephasing time to <1 μs, severely restricting the use of traditional CPBs in QIP. Engineering the CPB into the transmon regime E J ≫ E C (refs 17 , 18 ) exponentially suppresses the sensitivity of ω 01 to charge-parity and background charge fluctuations. However, recent theory [19] , [20] , [21] predicts that QP tunnelling remains a relevant source of relaxation and pure dephasing of the qubit degree of freedom. The contribution of QP tunnelling on qubit decoherence has become particularly interesting as control of the Purcell effect [22] in circuit quantum electrodynamics (cQED) [23] and the reduced contribution of dielectric losses in three-dimensional geometries [24] have allowed reaching the 100 μs scale. To guide further improvements, it is imperative to precisely pinpoint the timescale for QP tunnelling and its contribution to qubit decoherence. To date, only upper and lower bounds on QP tunnelling rates have been placed [18] , [25] in transmon qubits, while the effect of QP tunnelling on transmon decoherence remains unexplored. Here, we transform a state-of-the-art single-junction transmon qubit into a real-time charge-parity detector. We measure both the characteristic time for QP tunnelling across the junction and the effect of such tunnelling on qubit decoherence at the millisecond timescale. Our qubit is controlled and measured in a three-dimensional cQED architecture [24] , an emerging platform for QIP, without need for any electrometer or other circuitry. At the heart of our detection scheme is a very small but detectable parity dependence of the qubit transition frequency (up to 0.04% of the average ω 01 /2 π =4.387 GHz), obtained by choosing E J / E C =25. Evidence of QP tunnelling Standard Ramsey fringe experiments provide the first evidence of QP tunnelling across the qubit junction, as shown in Fig. 1 for a refrigerator temperature T r =20 mK. Instead of the usual single decaying sinusoid, we observe two. Repeated Ramsey experiments always reveal two frequencies, fluctuating symmetrically about the average ω 01 ( Fig. 1c ). The double frequency pattern results from QP tunnelling events causing n g to shift by ± e . The fluctuation in the difference Δ f between the two frequencies is owing to background charge motion slow compared with QP tunnelling. The observation of two frequencies in every experiment shows that QP tunnelling is fast compared with the averaging time ( ∼ 15 s), but slow compared with the maximum time 1/2Δ f ∼ 5 μs (ref. 26 ). From the similar amplitude of the sinusoids, we can already deduce that the two parities are equally likely. Clearly, these time-averaged measurements only loosely bound the timescale for QP tunnelling, similarly to refs 18 , 25 . 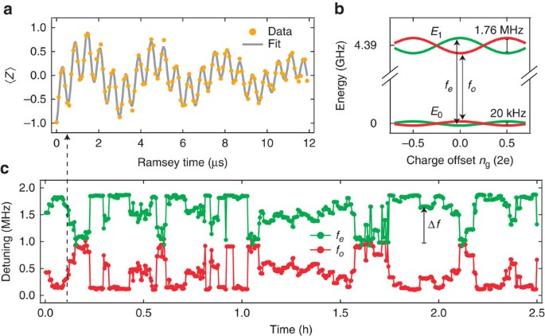Figure 1: Bistability and drift of the qubit transition frequency. (a) Ramsey fringe experiment (dots) and best-fit sum of two decaying sinusoids (curve). The reference oscillator is detuned 1 MHz from the average qubit transition frequencyω01/2π=4.387 GHz. (b) Sketch of the charge dispersion of the two lowest-energy levels of the transmon qubit, showing 2eperiodicity. QP tunnelling across the junction shiftsngby ±e, resulting in two transition frequenciesfeandfo(not to scale). (c) Repeated Ramsey experiments (15 s each) show a symmetric drift offeandfoaroundω01/2π, arising from background charge motion. The frequency difference 2Δf=fe−foranges from 0 to 1.76 MHz (see alsoSupplementary Fig. S1). Figure 1: Bistability and drift of the qubit transition frequency. ( a ) Ramsey fringe experiment (dots) and best-fit sum of two decaying sinusoids (curve). The reference oscillator is detuned 1 MHz from the average qubit transition frequency ω 01 /2 π =4.387 GHz. ( b ) Sketch of the charge dispersion of the two lowest-energy levels of the transmon qubit, showing 2 e periodicity. QP tunnelling across the junction shifts n g by ± e , resulting in two transition frequencies f e and f o (not to scale). ( c ) Repeated Ramsey experiments (15 s each) show a symmetric drift of f e and f o around ω 01 /2 π , arising from background charge motion. The frequency difference 2Δ f = f e − f o ranges from 0 to 1.76 MHz (see also Supplementary Fig. S1 ). Full size image Real-time detection of charge-parity fluctuations In order to accurately pinpoint the timescale for QP tunnelling, we have devised a scheme to monitor the charge parity in real time using the qubit itself ( Fig. 2a ). The scheme takes advantage of recent developments in high-fidelity nondemolition readout [27] , [28] and feedback control [29] . Starting from |0〉, the qubit is prepared in the superposition state ( with a π /2 y -pulse at ω 01 . The Rabi frequency of 16 MHz is sufficient to drive both odd- and even-parity qubit transitions, which differ by 2Δ f ≤1.76 MHz. The qubit then acquires a phase ± π /2 during a chosen idle time Δ t =1/4Δ f , where the + (−) sign corresponds to even (odd) parity. A second π /2 x -pulse completes the mapping of parity into a qubit basis state, even →|0〉, odd →|1〉. A following projective qubit measurement ideally matches the result P =1 (−1) to even (odd) parity. Feedback-based reset [29] reinitializes the qubit to |0〉 and allows repeating this sequence every Δ t exp =6 μs. 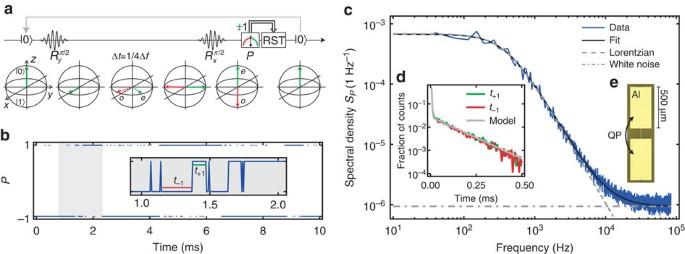Figure 2: Real-time measurement of QP tunnelling using the transmon qubit as its own charge-parity detector. (a) Ramsey-type sequence converting the qubit into a charge-parity detector. The sequence (see main text) is equivalent to a qubit flip conditioned on odd charge parity. (b) Snapshot (10 ms) of a typical measurement trace, 48 ms long, atTr=20 mK. Dots are repetitions of the experiment ina, at 6 μs interval. Inset: 1 ms zoom in, with indicated dwell timest+1andt−1forP=±1. (c) Double-sided power spectral density ofP, obtained by averaging the squared Fourier transform of 45 consecutive repetitions of (b). The best fit of equation (1) gives the QP tunnelling characteristic time 1/Γrts=0.794±0.005 ms and the overall detection fidelityF=0.918±0.002. Repeated experiments have a s.d. of 0.09 and 0.03 ms, respectively. (d) Histograms oft+1andt−1. The grey curve is a model of RTS, with ΓrtsandFextracted from the fit in the main panel. (e) Optical image of a qubit with identical geometry28to that used. SeeMethodsandSupplementary Figs S2–S4for several control experiments testing the measurement protocol. Figure 2: Real-time measurement of QP tunnelling using the transmon qubit as its own charge-parity detector. ( a ) Ramsey-type sequence converting the qubit into a charge-parity detector. The sequence (see main text) is equivalent to a qubit flip conditioned on odd charge parity. ( b ) Snapshot (10 ms) of a typical measurement trace, 48 ms long, at T r =20 mK. Dots are repetitions of the experiment in a , at 6 μs interval. Inset: 1 ms zoom in, with indicated dwell times t +1 and t −1 for P =±1. ( c ) Double-sided power spectral density of P , obtained by averaging the squared Fourier transform of 45 consecutive repetitions of ( b ). The best fit of equation (1) gives the QP tunnelling characteristic time 1/Γ rts =0.794±0.005 ms and the overall detection fidelity F =0.918±0.002. Repeated experiments have a s.d. of 0.09 and 0.03 ms, respectively. ( d ) Histograms of t +1 and t −1 . The grey curve is a model of RTS, with Γ rts and F extracted from the fit in the main panel. ( e ) Optical image of a qubit with identical geometry [28] to that used. See Methods and Supplementary Figs S2–S4 for several control experiments testing the measurement protocol. Full size image The time evolution of charge parity is encoded in the series of results P ( Fig. 2b ). The time series has zero average, confirming that the two charge parities are equally probable. Both the QP dynamics and the detection infidelity determine the distribution of dwell times t +1 and t −1 ( Fig. 2d ). The measured identical histograms match a numerical simulation of a symmetric random telegraph signal (RTS) with transition rate Γ rts , masked by uncorrelated detection errors occurring with probability (1− F )/2. These two noise processes contribute distinct signatures to the spectral density of P ( Fig. 2c ). The best fit of the form shows excellent agreement, giving 1/Γ rts =0.79 ms and F =0.92. Measurement of QP-tunnelling-induced qubit decoherence While the above scheme detects a characteristic time for QP tunnelling, our goal is to determine the effect of such QP tunnelling on the performance of the qubit degree of freedom. Specifically, we aim to determine the rates connecting level | kl 〉 to level | k ′ l ′〉 ( k ( k ′) and l ( l ′) denote the initial (final) qubit and parity state, respectively, as illustrated in Fig. 3b ). For example, denotes the QP-tunnelling-induced qubit relaxation rate. Based on the identical distribution of dwell times, we safely approximate symmetric rates . 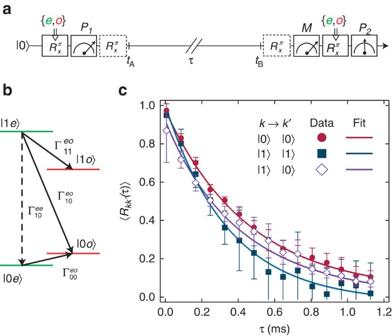Figure 3: Effect of QP tunnelling on the qubit degree of freedom. (a) Pulse sequence measuring the autocorrelation function of charge parity. Two charge-parity sequences, ending with measurementsP1andP2, respectively, are separated by a variable delay, followed by a qubit measurementM. We indicate by τ the time between the end ofP1and the start ofM. Postselection onP1=+1 (ref.28) prepares the state |0e〉. Similarly, a measurementM=+1 ensures that the final qubit state is |0〉.P2will coincide withP1only if the parity is unchanged. Insertingπrotations afterP1and/or beforeMallows measuring the parity autocorrelation for different combinations of qubit states. A preliminary measurement (not shown) initializes the qubit in |0〉 by postselection. Note that every measurement is projective on the qubit state. When the initial qubit state is known and the measurement is preceded by the parity-controlled qubit flip (Fig. 2), the result also denotes the charge parity. (b) Diagram of the four energy levels with the modelled transition rates (not to scale). (c) Charge-parity autocorrelationRkk′(τ) for qubit in state |0〉 (dots), |1〉 (squares), or having relaxed from |1〉 to |0〉 (diamonds) during τ (Tr=20 mK). The average of the conditionedP2is corrected for detection infidelity (seeMethods). Fitting the solution of the rate equations, conditioned on initial and final qubit states, gives the inverse rates:,,,. Figure 3: Effect of QP tunnelling on the qubit degree of freedom. ( a ) Pulse sequence measuring the autocorrelation function of charge parity. Two charge-parity sequences, ending with measurements P 1 and P 2 , respectively, are separated by a variable delay, followed by a qubit measurement M . We indicate by τ the time between the end of P 1 and the start of M . Postselection on P 1 =+1 (ref. 28 ) prepares the state |0 e 〉. Similarly, a measurement M =+1 ensures that the final qubit state is |0〉. P 2 will coincide with P 1 only if the parity is unchanged. Inserting π rotations after P 1 and/or before M allows measuring the parity autocorrelation for different combinations of qubit states. A preliminary measurement (not shown) initializes the qubit in |0〉 by postselection. Note that every measurement is projective on the qubit state. When the initial qubit state is known and the measurement is preceded by the parity-controlled qubit flip ( Fig. 2 ), the result also denotes the charge parity. ( b ) Diagram of the four energy levels with the modelled transition rates (not to scale). ( c ) Charge-parity autocorrelation R kk ′ (τ) for qubit in state |0〉 (dots), |1〉 (squares), or having relaxed from |1〉 to |0〉 (diamonds) during τ ( T r =20 mK). The average of the conditioned P 2 is corrected for detection infidelity (see Methods ). Fitting the solution of the rate equations, conditioned on initial and final qubit states, gives the inverse rates: , , , . Full size image To extract the above rates, we measure the autocorrelation function of charge parity, conditioned on specific initial and final qubit states ( Fig. 3 ). We first execute the charge-parity sequence illustrated in Fig. 2 . Conditioning on the result of the projective measurement P 1 =+1 postselects the qubit in |0〉 and even parity. After a waiting time τ , another measurement M determines the qubit state. Conditioning also on M =+1 ensures that the qubit ends in |0〉. A second instance of the charge-parity sequence, ending with P 2 , completes the scheme. The average result, once corrected for detector infidelity (see Methods ), is the parity autocorrelation R 00 ( τ )=〈 P (0) P ( τ )〉 00 , with first (second) subscript indicating initial (final) qubit state. Neglecting qubit excitation, that is, setting , R 00 (τ) simply decays as . The exact solution shows that this remains a valid approximation when including the measured Γ 01 =1/6 ms −1 , as the probability of multiple qubit transitions in τ is negligible. Similarly, we measure the parity autocorrelation with qubit initially and finally in |1〉, . To do this, we use the same conditioning, but apply a π pulse after P 1 and before M . Exponential decay fits give and . To quantify the contribution of QP tunnelling to the measured net qubit relaxation time T 1 =1/Γ 10 =0.14±0.01 ms (see Methods ), we apply the same method, but condition on initial state |1〉 and final state |0〉. The ratio of QP-induced to total relaxation rates can be extracted from R 10 (τ→0)=1−2 α . The best fit of the model R 10 (τ) to the data, with α as only free parameter, gives and . This result clearly demonstrates that QP tunnelling does not dominate qubit relaxation at T r =20 mK, contributing only 5% of qubit relaxation events. To facilitate comparison of the measured rates to theory, we perform the above experiments at elevated T r ( Fig. 4 ). We observe that , and have similar magnitude and jointly increase with T r in the range 20–170 mK. However, T 1 remains insensitive to T r until 150 mK. The observed sign reversal in R 10 (τ→0) near this temperature ( Fig. 4b ) indicates that QP tunnelling becomes the dominant qubit relaxation process. 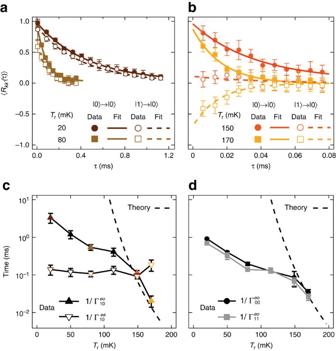Figure 4: Temperature dependence of QP tunnelling contribution to qubit relaxation and dephasing. (a,b) Charge-parity autocorrelation functionsR00(τ) andR10(τ) at 20,80 (a), 150 and 170 mK (b).R10(τ→0) progressively decreases, indicating an increasing contribution of QP tunnelling to qubit relaxation. (c) Relaxation times with (, upward triangles) and without (, downward triangles) QP tunnelling, obtained fromR10(τ). Dashed curve: equation (2) for thermal equilibrium. (d) Times for QP tunnelling times without qubit relaxation in the ground-state (, dots) and excited-state (, squares) manifold extracted fromR00(τ) andR11(τ) (not shown). Dashed curve: theory for(refs19,21) for thermally distributed QPs and Δ=170 μeV. Error bars are 1 s.d. SeeSupplementary Fig. S5for the temperature dependence of Γrts. Figure 4: Temperature dependence of QP tunnelling contribution to qubit relaxation and dephasing. ( a , b ) Charge-parity autocorrelation functions R 00 (τ) and R 10 (τ) at 20,80 ( a ), 150 and 170 mK ( b ). R 10 (τ→0) progressively decreases, indicating an increasing contribution of QP tunnelling to qubit relaxation. ( c ) Relaxation times with ( , upward triangles) and without ( , downward triangles) QP tunnelling, obtained from R 10 (τ). Dashed curve: equation (2) for thermal equilibrium. ( d ) Times for QP tunnelling times without qubit relaxation in the ground-state ( , dots) and excited-state ( , squares) manifold extracted from R 00 (τ) and R 11 (τ) (not shown). Dashed curve: theory for (refs 19 , 21 ) for thermally distributed QPs and Δ=170 μeV. Error bars are 1 s.d. See Supplementary Fig. S5 for the temperature dependence of Γ rts . Full size image The effect of QP dynamics on the qubit degree of freedom in superconducting circuits has been extensively studied theoretically [7] , [19] , [20] , [21] . For transmon qubits, the predicted QP-induced relaxation rate is [19] , [20] where x qp = n qp /2 ν 0 Δ is the QP density n qp normalized to the Cooper-pair density, with ν 0 =1.2 × 10 4 μm −3 μeV −1 the single-spin density of states at the Fermi energy [11] and Δ the Al superconducting gap. This relation holds for any energy distribution of QPs. For T r ≥150 mK, the data closely match equation (2) using the thermal equilibrium and Δ=170 μeV, the value estimated from the normal-state resistance of the junction (see Methods ). The suppression of at lower T r is much weaker than expected from a thermal QP distribution. Using equation (2), we estimate n qp =0.04±0.01 μm −3 at T r =20 mK, matching the lowest value reported for Al in a Cooper-pair transistor for use in metrology [30] . Improved shielding against infrared radiation [31] could further decrease n qp at low T r , consequently suppressing the contribution of QP tunnelling to qubit relaxation, and will be pursued in future work. QP tunnelling events that do not induce qubit transitions still contribute to pure qubit dephasing. Calculations based on refs 19 , 21 predict , in good agreement with the data ( Fig. 4c ). It is presently not understood whether such QP tunnelling events completely destroy qubit superposition states (case A) or simply change the qubit precession frequency (case B). In either case, in the regime of strongly coupled RTS valid for our experiment ( (ref. 26 )) the QP-induced dephasing time is . For case B, this time would further increase in the weak-coupling regime (attained at E J / E C ≳ 60) owing to motional averaging [26] . In conclusion, we have converted a state-of-the-art transmon qubit into its own charge-parity detector to answer whether QP tunnelling already limits qubit coherence. We measure the contribution of QP tunnelling to relaxation and dephasing to be in the millisecond range. We stress that these times are directly measured, without relying on any theory. Thus, transmon qubit coherence can increase by at least another order of magnitude before QP tunnelling begins to limit coherence. Such an increase would facilitate the realization of fault-tolerant quantum computing in the solid state. The implemented scheme also provides an essential ingredient in the envisioned top-transmon architecture for manipulation and readout of Majorana qubits [32] . Device parameters The transmon has Josephson energy E J =8.442 GHz and charging energy E C =0.334 GHz. Using the Ambegaokar–Baratoff relation E J R n =Δ/8 e 2 and the measured room-temperature resistance R n,300K =15.2 kΩ of the single Josephson junction, we estimate Δ=170 μeV. The qubit couples to the cavity fundamental mode ω r /2 π =6.551 GHz (decay rate κ /2 π =720 kHz) with strength g /2 π =66 MHz, inducing a dispersive shift χ / π =−1.0 MHz. The qubit relaxation time T 1 may be limited by the multi-mode Purcell effect [22] . A simple estimate including only the fundamental mode gives 240 μs. The dephasing time, μs, is limited by background charge fluctuations (see Supplementary Fig. S1 ). Experimental setup The device and the experimental setup are similar to those described in refs 28 , 29 . Here, we detail the changes we made since these earlier reports. In an effort to lower the transmon residual excitation, we replaced the Al cavity with a Cu cavity [33] , improved thermal anchoring to the mixing chamber plate and added low-pass filters (K&L Microwave 6L250-8000/T18000-O/O) on the input and output ports of the cavity. As a result, the transmon effective temperature decreased from 127 to 55 mK, corresponding to a reduction of total steady-state excitation from ∼ 16 to 2%, respectively. As these changes were made simultaneously, we cannot pinpoint the individual contributions to the improved thermalization.Projective readout with 99% fidelity is achieved by homodyne detection with a 400 ns pulse at ω r − χ , aided by a Josephson parametric amplifier [28] . To perform qubit reset faster, we replaced the ADwin processor with a home-built feedback controller based on a complex programmable logic device (CPLD, Altera MAX V). The CPLD integrates the last 200 ns of the readout signal and conditionally triggers a π pulse (all resonant pulses are Gaussian, with σ =8 ns, and total duration 32 ns). The CPLD allows a response time, from the end of signal integration to the π -pulse trigger, of 0.11 μs. The total loop time, from the start of the measurement pulse to the end of the triggered π pulse at the cavity input, is 0.98 μs. However, a delay is added to reach 2 μs ( ∼ 10/ κ ) between the end of measurement and the start of the conditioned π pulse, ensuring that the cavity is devoid of readout photons. Extraction of QP tunnelling rates To convert 〈 P 2 (τ)〉 kk ′ into R kk ′ (τ), we correct for the overall detection errors, distributed among readout (<1%) and reset ( ∼ 1%) infidelities, suboptimal Δ t (<2%) and dephasing during Δ t (remaining 1−3%). For this correction, we first fit an exponential decay to 〈 P 2 (τ)〉 00 and 〈 P 2 (τ)〉 11 . The average of the best-fit value at τ =0 is used to renormalize the data in Figs 3c and 4a . The fitted decay times are and , respectively. To extract and , we fit the solution of equation (2) to R 10 (τ), using . Γ 10 is obtained from the equilibration time T eq after inverting the steady-state populations P |0〉,ss , P |1〉,ss with a π pulse: The total excitation 1− P |0〉,ss is obtained by measurement and postselection [29] . Equation (3) remains a valid approximation even for the highest temperatures in Fig. 4 , at which population of higher excited states becomes relevant. In this case, the populations P |0〉,ss , P |1〉,ss are estimated from the total excitation, assuming that the populations are thermally distributed [29] . Error bars for are calculated from the s.d. of repeated T 1 measurements and the fit uncertainty in α . Validation of the charge-parity detector We perform several control experiments to validate the use of the qubit as a charge-parity detector. First, the parity to qubit-state conversion is tested with suboptimal choices of the Ramsey interval Δ t ( Supplementary Fig. S2 ). As expected from equation (1), the white noise level in S P increases at the expense of the signal contrast as Δ t deviates from the optimal choice 1/4Δ f . Remarkably, the extracted rate Γ rts is approximately constant down to F ∼ 0.4. This is consistent with the model of charge parity as a symmetric RTS, with time constant determined solely by QP tunnelling.In a second test, we replace the Ramsey-like sequence with a single pulse, with rotation angle θ . Time series of M for θ =0, π and π /2 are shown in Supplementary Fig. S3a . The very high occurrence ( ∼ 99%) of 1 (−1) for θ =0 ( π ) equals the efficiency of reset, following each measurement M . For θ = π /2, the qubit is repeatedly prepared in an equal superposition of |0〉 and |1〉, and the measurement produces uncorrelated projection noise. The spectra of these control experiments are compared with the QP tunnelling measurement in Supplementary Fig. S3b , clearly showing that the observed RTS is owing to the signal acquired during Δ t .As a final test of the charge-parity detector, we subject the qubit to an externally generated RTS, similar to ref. 25 . Symmetric RTS sequences with switching rate Γ π are generated in LabVIEW and sent to an ADwin controller. The ADwin samples the RTS at 9 μs interval. When the signal is +1, the ADwin triggers an AWG520 (also used for reset [29] ), which then applies a π pulse on the qubit. As a result, the measured qubit state in M is conditioned on the RTS state, mimicking the parity-controlled π pulse implemented in Fig. 2 . In all cases, the fitted rates Γ fit match the programmed Γ π within 3% ( Supplementary Fig. S4 ). How to cite this article: Ristè, D. et al . Millisecond charge-parity fluctuations and induced decoherence in a superconducting transmon qubit. Nat. Commun. 4:1913 doi: 10.1038/ncomms2936 (2013).